Interleukin-7 receptor α mutational activation can initiate precursor B-cell acute lymphoblastic leukemia 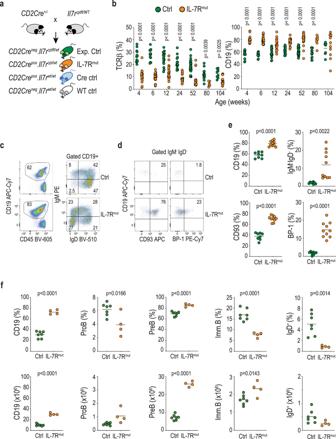Fig. 1: Physiological levels of heterozygous mutant IL-7Rα expression consistently originate a B cell precursor pre-leukemic stage. aScheme of experimental cross, depicting genotype of progeny. Green (controls) and orange (IL-7Rmut) animals were bled from week 4 and monitored up to week 104, unless disease ensued. A cohort of Cre-toxicity controls (blue) was also monitored that presented no disease.bTCRβ and CD19 fractions within CD45-positive cells in blood from control and IL-7Rmutanimals. Each dot denotes an animal and mean value is shown. Two-tailed unpairedt-test.cCD19 fraction (left) and IgM versus IgD subpopulations within CD19 (right) in the blood of one representative animal from each group at 6 weeks of age. Numbers indicate frequencies of each quadrant or region.dCD93 and BP-1 expression within IgM−IgD−cells in the blood from the same animals than inc.eScatter plots summarizing data from all animals analyzed as incandd. Ctrls:n= 8; IL-7Rmut:n= 10. Each dot denotes an animal and mean value is shown. Two-tailed unpairedt-test.fScatter plots showing fractions (top) and absolute numbers (bottom) in BM for the indicated populations in 4-week-old animals from Ctrl (n= 7) and IL-7Rmut(n= 4) animals. Two-tailed unpairedt-test. Source data are provided as a Source Data file. Interleukin-7 receptor α (encoded by IL7R ) is essential for lymphoid development. Whether acute lymphoblastic leukemia (ALL)-related IL7R gain-of-function mutations can trigger leukemogenesis remains unclear. Here, we demonstrate that lymphoid-restricted mutant IL7R , expressed at physiological levels in conditional knock-in mice, establishes a pre-leukemic stage in which B-cell precursors display self-renewal ability, initiating leukemia resembling PAX5 P80R or Ph-like human B-ALL. Full transformation associates with transcriptional upregulation of oncogenes such as Myc or Bcl2 , downregulation of tumor suppressors such as Ikzf1 or Arid2 , and major IL-7R signaling upregulation (involving JAK/STAT5 and PI3K/mTOR), required for leukemia cell viability. Accordingly, maximal signaling drives full penetrance and early leukemia onset in homozygous IL7R mutant animals. Notably, we identify 2 transcriptional subgroups in mouse and human Ph-like ALL, and show that dactolisib and sphingosine-kinase inhibitors are potential treatment avenues for IL-7R-related cases. Our model, a resource to explore the pathophysiology and therapeutic vulnerabilities of B-ALL, demonstrates that IL7R can initiate this malignancy. Acute lymphoblastic leukemia (ALL), the most common childhood malignancy, is an aggressive cancer arising from lymphoid progenitors, especially of the B lineage [1] . Although current therapies are highly effective, with 5-year survival rates reaching 80–90%, a significant number of ALL cases still relapse and the use of intensive chemotherapy has substantial short- and long-term side effects, including decreased life expectancy [1] , [2] . Importantly, therapeutic success in adults lags significantly behind, with only 30–40% of the cases surviving long term [3] . As such, improving the understanding of ALL molecular causes and underlying biology is critical to better classify patients and identify the best targeted treatment options that can improve efficacy and minimize toxicities for each particular patient subset. The axis constituted by interleukin-7 (IL-7) and its receptor (IL-7R), composed of IL-7Rα (encoded by IL7R ) and γc (encoded by IL2RG ), is essential for normal lymphoid development—its inactivation resulting in severe combined immunodeficiency [4] , [5] , [6] , [7] . During B cell development, IL-7Rα signaling is tightly regulated and, together with the pre-BCR, sequentially coordinates proliferation and Ig gene rearrangements, in cross-talk with critical transcription factors such as PAX5, EBF1 or IKAROS [8] , [9] . The importance of keeping IL-7R-mediated signaling under control is illustrated by studies showing that Il7 transgenic mice develop B cell lymphomas, and that IL-7 induces proliferation of human B-ALL cells [7] . Moreover, B-ALL arising in Pax5 -deficient mice exposed to infection [10] or in mice with combined loss of Sh2b3 and Trp53 (ref. [11] ) involves an IL-7 hypersensitive pre-leukemic stage, and IL-7Rα is required for B-ALL developing in mice from the combination of Stat5 activation and Pax5 haploinsufficiency [12] . Somatic IL7R gain-of-function mutations were identified in around 10% of T-ALL cases and in B-ALL [13] , [14] , where they are enriched in particular subgroups, including Ph-like and PAX5 P80R B-ALL [15] , [16] , [17] , [18] , [19] . Studies relying on retroviral transduction of mouse hematopoietic progenitors or thymocytes and subsequent transplantation into recipient mice showed that overexpression of mutant IL-7Rα can collaborate with other oncogenic insults ( Cdkn2a deletion, NRAS G13D mutation, and intracellular NOTCH1 overexpression) to promote T-ALL [20] , [21] , [22] . These studies, however, did not separate the effect of IL7R mutation from IL7R overexpression, and were conducted in the context of already compromised hematopoiesis (in immunodeficient or irradiated recipient mice). Moreover, ectopic IL7R expression can considerably bias the results, as illustrated by mutant IL-7Rα resulting in myeloid neoplasia or IgM-positive mature B cell leukemia/lymphoma [22] , for which no IL7R mutations have been reported in humans. Thus, it remains unclear whether mutational activation of IL-7Rα without concomitant overexpression, can effectively trigger ALL, i.e., whether IL7R mutations per se can be the initiating event. This is particularly relevant because it is commonly accepted that ALL is triggered by fusions (such as BCR-ABL1, ETV6-RUNX1 or those involving KMT2A) resulting from chromosomal rearrangements [23] , or by lesions affecting transcription factors (such as PAX5 P80R) [16] , but there is no clear evidence that gain-of-function mutations in signaling-related genes can initiate ALL. Here, we generated and characterized a conditional knock-in model in which mutant IL-7Rα is expressed at physiological levels from the common lymphoid progenitor (CLP) stage. We demonstrate that IL7R gain-of-function is sufficient to trigger leukemogenesis leading to the development of PAX P80R or Ph-like precursor B-ALL with high penetrance, reflecting the enrichment in these two subtypes within IL7R mutant human cases. We find that IL7R-dependent Ph-like ALL in the mouse subdivides into two subgroups with distinct transcriptional and mutational signatures that also exist in human cases. Subsequent hits potentially contributing to leukemia development affect genes known to be involved in human B-ALL (e.g Pax5 , Trp53 , Kras ) as well as new candidates (e.g Limk1 , Cdc42bpb ). We further show that Kras mutation cooperates with IL7R mutation in upregulating IL7R-mediated signaling in pre-leukemic cells. In addition, leukemias display transcriptional upregulation of oncogenes such as Myc or Bcl2 , and downregulation of tumor suppressors such as Ikzf1 , Ikzf2 , Arid1b , or Arid2 . Irrespective of the collaborating hits, the transformation process clearly associates with a striking increase in IL-7R-mediated signaling (evidenced e.g. by mTOR and STAT5 signaling upregulation, as well as MYC activation) from the pre-leukemic to the leukemic stage, and IL-7R-mediated signaling is required for leukemia cell maintenance. Homozygous IL7R mutant mice, which show maximal signaling, develop very rapid, fatal leukemia with a trend for lower mutational burden, thereby illustrating the importance of IL-7R signaling upregulation in driving leukemogenesis. Finally, we use our model and human patient samples to demonstrate that PI3K/mTOR and sphingosine kinase inhibitors may constitute valid therapeutic approaches to treat IL7R mutant ALL cases. Physiological levels of heterozygous mutant IL-7Rα expression consistently originate a B cell precursor pre-leukemic stage Although some B-ALL cases harbor clonal IL7R gain-of-function mutations [15] , [16] , suggesting that IL7R activation can be an early event in leukemia development, there is no formal evidence that IL7R drives B-ALL. Moreover, studies addressing the leukemogenic potential of IL7R gain-of-function mutations relied on retroviral overexpression and subsequent transplantation into immunocompromised mice [20] , [21] , [22] . To more rigorously evaluate the capacity of mutant IL-7Rα to transform B cell precursors in vivo and to originate B-ALL, we first introduced a human type 1a mutant IL7R form [7] , [13] into the mouse coding sequence and validated its ability to promote constitutive signaling and to transform Ba/F3 cells (Supplementary Fig. 1 ). Then, using a FLEx switch strategy, we generated conditional mutant IL7R knock-in mice (Supplementary Fig. 2 ) that we crossed with CD2-Cre animals (Fig. 1a ) to produce progeny in which recombination occurs at the CLP stage [24] , allowing for physiological regulation of mutant IL7R expression in developing lymphoid cells. The preservation of the normal developmental patterns of IL-7Rα modulation in our model is best illustrated during thymic T cell differentiation, where IL-7Rα expression levels are tightly and dynamically regulated (Supplementary Fig. 3 ). Our strategy prevented mutant IL7R overexpression (Supplementary Fig. 4 ) and abnormal surface IL-7Rα upregulation (Supplementary Fig. 5 ), ensuring that putative functional impacts were strictly due to IL7R mutational activation. Fig. 1: Physiological levels of heterozygous mutant IL-7Rα expression consistently originate a B cell precursor pre-leukemic stage. a Scheme of experimental cross, depicting genotype of progeny. Green (controls) and orange (IL-7R mut ) animals were bled from week 4 and monitored up to week 104, unless disease ensued. A cohort of Cre-toxicity controls (blue) was also monitored that presented no disease. b TCRβ and CD19 fractions within CD45-positive cells in blood from control and IL-7R mut animals. Each dot denotes an animal and mean value is shown. Two-tailed unpaired t -test. c CD19 fraction (left) and IgM versus IgD subpopulations within CD19 (right) in the blood of one representative animal from each group at 6 weeks of age. Numbers indicate frequencies of each quadrant or region. d CD93 and BP-1 expression within IgM − IgD − cells in the blood from the same animals than in c . e Scatter plots summarizing data from all animals analyzed as in c and d . Ctrls: n = 8; IL-7R mut : n = 10. Each dot denotes an animal and mean value is shown. Two-tailed unpaired t -test. f Scatter plots showing fractions (top) and absolute numbers (bottom) in BM for the indicated populations in 4-week-old animals from Ctrl ( n = 7) and IL-7R mut ( n = 4) animals. Two-tailed unpaired t -test. Source data are provided as a Source Data file. Full size image As early as 4 weeks, IL7R mutant (CD2Cre Pos .Il7r cpt/wt ) mice displayed decreased T cell and increased B cell frequency in the blood (Fig. 1b ). Although T cell precursors expressed mutant IL7R transcript levels similar to those of B cell precursors (Supplementary Fig. 6 ) there was no major impact on T cell development in the thymus (Supplementary Fig. 7 ), or on the distribution of mature T lymphocyte subpopulations (Supplementary Fig. 8 ). Instead, IL7R mutation affected the B cell lineage leading to aberrant frequency of IgM − IgD − CD93 + BP-1 + B cell precursors in the blood (Fig. 1c–e ) that resulted from a major expansion of B cell precursors in the bone marrow (BM) (Fig. 1f ). This pre-leukemic phenotype, characterized by partial differentiation arrest and expansion of pro- and pre-B cells, affected all CD2Cre Pos .Il7r cpt/wt mice. Pre-leukemic cells had higher viability, but not proliferation, than normal B cell precursors (Supplementary Fig. 9 ) and displayed enrichment in stemness genes and increased self-renewal potential, in some cases leading to leukemia development upon transfer into recipient mice (Supplementary Fig. 10 ). Mutant IL-7Rα drives B-ALL The pre-leukemic stage eventually evolved into overt fatal leukemia in a majority of the mice (Fig. 2a ), with high penetrance (reaching > 60% at 80 weeks) and a median latency of 43 weeks and a range of 8 to >90 weeks. This broad range resembles that described in humans, where ALL patients of different ages (children, adolescents, and adults) can display IL7R mutations. In addition to the BM, leukemia cells spread to the spleen, kidney, liver, lung, and CNS (Fig. 2b ). In contrast to control and pre-leukemic cells, leukemias were clonal, as assessed by analysis of Ig gene rearrangements (Fig. 2c and Supplementary Fig. 11 ), displayed a higher IgH/(κ + λ) ratio (Fig. 2d ) than pre-leukemias and normal controls, and had a gene expression profile closer to that of pro- and pre-B cell precursors than of mature splenic B cells (Fig. 2e ). In agreement, their maturation arrest ranged from early pro-B to the small pre-B cell stage (Fig. 2f and Supplementary Data 1 ), altogether indicating they corresponded to bona fide precursor B-ALL. In accordance, the V(D)J rearrangements of the major clone(s) in each leukemia were productive in some cases (e.g. #2672 and #13573, both arrested at the small pre-B cell stage) and non-productive in others (e.g. #2674, a pro-B cell leukemia; Supplementary Data 2 ). Leukemias were transplantable (Fig. 2g ) and leukemia-propagating cells were IgM − IgD − (Fig. 2h ). As expected from IL-7R-driven tumors [25] , [26] , leukemic cells displayed high Myc and Bcl2 levels (Fig. 2i ), and higher proliferation (Fig. 2j ) and viability (Fig. 2k ) than normal and pre-leukemic B cell precursors. Moreover, they presented distinctive transcriptional (Fig. 3a and Supplementary Data 3–4) and protein (Fig. 3b and Supplementary Data 5 and 6 ) expression profiles, with enrichment for ribosome, oxidative phosphorylation, and spliceosome pathways (Supplementary Fig. 12 ). Transcriptome and proteome data integration confirmed the enrichment for ribosome biogenesis, as well as RNA transport and different metabolic pathways, including cysteine and methionine metabolism, amino sugar and nucleotide sugar metabolism, carbon metabolism (Fig. 3c ), and cholesterol homeostasis (Fig. 3d ). Moreover, we found an enrichment for unfolded protein response (Fig. 3e ), which has been proposed as a valid therapeutic target in B-ALL [27] . Fig. 2: IL-7Rα mutant mice develop precursor B-ALL. a Example of IgM − IgD − cell frequency evolution in a mouse that developed leukemia (top). Kaplan–Meier leukemia-free survival curves of control (Ctrl; n = 40) and IL7R mutant (IL7R mut ; n = 63) animals (bottom). All mice died with precursor B-ALL. Log-rank Mantel–Cox test ( b ) Histologies (H&E) of organs infiltrated with leukemia cells. Pie chart inserts represent fraction of analyzed animals ( n = 4) with leukemia involvement (in black) in the respective organ. Scale bar indicates 100 μm (bone marrow, spleen), 250 μm (kidney, lung, liver), or 500 μm (brain). c Clonality pie charts based on IgH sequencing. Each colored slice corresponds to a clone, indicative of clonality. Gray areas correspond to many rare clones, indicative of polyclonality. Equitability values (ranging from 0, for monoclonality, to 1, for a balanced repertoire) are shown in the center of the pie charts. Samples are bone marrow pro+pre-B cells from control, pre-leukemic, or leukemic mice. d Ig heavy chain (H) over light chain (κ and λ) ratios to evaluate, at the population level, the presence of the pro-B cell rearrangement signature (heavy chain expression in the absence of light chain expression). Two-tailed Mann–Whitney test performed. e Principal component analysis of normal (Ctrl Pro+Pre-B) and pre-leukemic (Pre-leukemic) pro- and pre-B cell precursors, mature splenic B cells (Ctrl IgD + ) and leukemia cells (IL7R mut Leuk). f Immunophenotypic analysis of three representative BM leukemia samples. Numbers inside dot plots indicate frequency in each quadrant or region. g , h Kaplan–Meier leukemia-free survival curves of mice transplanted with g bulk primary leukemias or h sorted IgD + versus IgM − IgD − leukemia cells. i Myc and Bcl2 transcript upregulation (log2 fold change) in leukemia samples ( n = 9) as compared to normal controls ( n = 5). Moderated t -test performed. j Frequency of Ki67-positive cells in controls ( n = 5), pre-leukemia ( n = 5), and leukemia samples ( n = 5). Dot plots are representative of each condition. k Frequency of annexin V/7AAD-negative (viable) cells in controls ( n = 9) pre-leukemia ( n = 8) and leukemia samples ( n = 9). Dot plots are representative of each condition. j , k Two-tailed unpaired t -test. Source data are provided as a Source Data file. Full size image Fig. 3: Transcriptomics and proteomics characterization of mutant IL7R leukemias. a Heatmap representation and hierarchical clustering of control and leukemia samples based on the 1000 most significant (adj. p value) differentially expressed genes. b Heatmap representation of samples based on the 500 most significant (nominal p value) differentially expressed proteins between control and leukemia samples. c g:Profiler KEGG pathway functional enrichment analysis for significant and concordantly upregulated genes and proteins in leukemia samples. Significantly enriched pathways (A–G, adj. p < 0.05. Cumulative hypergeometric test) are represented in full opacity. Pathways below the significance threshold are represented in low opacity. Pathways where p = 1 are not featured. d , e Gene set enrichment analysis (GSEA)-enrichment plot of differential gene and protein expression between leukemias and controls showing a significant upregulation of the d cholesterol homeostasis and the e unfolded protein response (UPR) hallmark gene sets (normalized enrichment score (NES) > 1, FDR < 0.05). Source data are provided as a Source Data file. Full size image Leukemic transformation of B cell precursors downstream from IL7R mutation associates with upregulation of IL-7R-mediated signaling activation We next sought to document IL-7R-mediated signaling alterations during the transformation process. Since healthy developing B lymphoid precursors are exposed to IL-7 in vivo, we cultured ex vivo pre-leukemic and normal B cell precursors in the absence of IL-7 to expose cell-intrinsic differences. We confirmed that pre-leukemia cells displayed cell-autonomous upregulation of IL-7R-mediated signaling, measured by phospho-STAT5 and phospho-S6 levels (Fig. 4a ). In vivo, IL-7R signaling pathway target genes were mildly upregulated in pre-leukemia cells as compared to normal controls (Fig. 4b ). However, leukemia establishment associated with marked IL-7R signaling upregulation (Fig. 4b ). This was reflected in the activation of key downstream targets [26] , [28] , [29] , [30] , [31] , such as STAT5 (Fig. 4c ), MYC (Fig. 4d and Supplementary Fig. 13 ), and mTOR (Fig. 4e–g ). Accordingly, gene set enrichment analysis of pre-leukemic versus control samples showed several significantly upregulated pathways, including cholesterol homeostasis and the unfolded protein response, metabolism-related pathways (e.g. glycolysis, fatty acid metabolism, oxidative phosphorylation), and signaling pathways (MYC, PI3K/mTOR), which were further upregulated in leukemic mice (Supplementary Fig. 14 ). These observations align with IL-7R-mediated signaling increasing from control to pre-leukemia and then further augmenting upon conversion to leukemia. Importantly, leukemia cell viability relied on maintenance of high IL-7R-mediated signaling, as shown by inhibition of JAK1, STAT5, or PI3K/mTOR signaling (Fig. 4h ), or by the use of the bromodomain inhibitor JQ1 to concomitantly target IL7R and MYC transcriptionally [32] (Supplementary Fig. 15 ). Fig. 4: Leukemia cells rely on IL-7R signaling, which boosts upon transformation. a Immunoblot analysis of phosphorylated STAT5 and S6 levels in sorted pro+pre-B cells from control ( n = 4) and pre-leukemic ( n = 3) mice, IL-7-deprived for 12 h. Graphs represent densitometry values for P-STAT5 and P-S6 normalized to respective total protein. b Differential gene expression of known IL-7R signaling targets in pre-leukemia and leukemia samples compared to controls (reference category). Moderate t -test performed. c – e Differential expression of ( c ) STAT5, ( d ) MYC, and ( e ) mTOR targets in leukemia versus control samples. Significantly upregulated and downregulated genes (adj. p < 0.05; moderate t -test) are shown in red and in blue, respectively. f Immunoblot analysis of phosphorylated S6 levels in control ( n = 3) and leukemia ( n = 6) samples analyzed ex vivo. g Transcriptomic and proteomic gene set enrichment analysis (GSEA) showing a significant enrichment of the mTOR signaling hallmark gene set in leukemias versus controls. h Leukemia cells were cultured in the presence or absence of pharmacological inhibitors of JAK1/2 (INCB018424; ruxolitinib), STAT5 (STAT5 inhibitor), and PI3K (LY294002) at the indicated doses, and viability was evaluated at 48 and 72 h. Results from a representative mouse ( n = 3). Lines represent average of duplicates that are shown. Source data are provided as a Source Data file. Full size image Homozygous expression of mutant IL7R leads to early disease onset and full penetrance These observations suggested there was a strong selective advantage for B cell precursors to display high levels of IL-7R-mediated signaling on the path leading to leukemia development. If so, maximal IL-7R signaling should drive faster leukemia development. In agreement, homozygous expression of mutant IL7R in CD2Cre Pos .Il7r cpt/cpt mice led to early accumulation of B cell precursors in the blood (Fig. 5a ), rapidly followed by precursor B-ALL establishment (Fig. 5b, c , Supplementary Fig. 16 and Supplementary Data 1 ). Leukemia developed with very rapid kinetics (median latency of 12 weeks) and full penetrance at 31 weeks (Fig. 5b ), and displayed highest IL-7R-mediated signaling levels (Fig. 5d and Supplementary Figs. 16 and 17 ). Leukemias from IL7R mutant homozygous mice were polyclonal (Fig. 5e ) and tended to have less mutational burden, including of high and moderate impact variants (Supplementary Fig. 17 ) than those from IL7R heterozygous animals, suggesting that highest IL-7R signaling levels easily transform B cell precursors without requiring (a large number of) additional oncogenic hits. Overall, these results indicate that transformation downstream of IL7R mutational activation converges on the potentiation of IL-7R signaling itself and stronger activation overcomes more efficiently the barriers to B-ALL development. Fig. 5: Homozygous expression of mutant IL7R leads to maximal IL-7R signaling hyperactivation and rapidly fatal leukemia. a Dot plots of CD19 by TCRβ to identify T and B cell lymphocytes in blood at 6 weeks of age in representative animals of indicated genotypes (left) and graphs summarizing data from all animals analyzed (right). Ctrls: n = 8; IL-7R mut Het: n = 10; IL-7R mut Hom: n = 5. Each dot denotes an animal and mean value is shown. Numbers in dot plots indicate frequency in each quadrant. One-way ANOVA. b Kaplan–Meier leukemia-free survival curves of control ( n = 40), IL-7R mut Het ( n = 63), and IL-7R mut Hom ( n = 20) mutant animals. Log-rank (Mantel–Cox) test. All mice died with precursor B-ALL. c Immunophenotypic analysis of three representative BM IL-7R mut Hom leukemia samples. Numbers inside dot plots indicate frequency in each quadrant or region. d Comparison of IL-7R “signaling strength” between IL-7R mut Het and IL-7R mut Hom leukemia samples, as measured by the levels of differential gene expression over control samples. Each dot represents log2 fold change (FC) of an IL-7R signaling target gene (see Fig. 4b ). Means are indicated. Unpaired two-tailed t -test. e Clonality pie charts based on IgH sequencing (see Fig. 2c for further details). Source data are provided as a Source Data file. Full size image Mutant IL7R leads to the development of PAX5 P80R and Ph-like ALL A considerable fraction of human B-ALL cases from particular subtypes, especially PAX5 P80R and Ph-like, harbor IL7R mutations [16] . This raises the possibility that mutant IL7R may drive preferentially certain types of precursor B-ALL. In agreement, centroid analysis of the gene expression profile of IL7R mutant mouse tumors revealed they resemble precisely PAX5 P80R or Ph-like human B-ALL (Supplementary Data 7 ). Principal component analysis (PCA) confirmed the existence of two subgroups, which discriminated the cases identified as PAX5 P80R or Ph-like (Fig. 6a ). Notably, whole-exome sequencing (WES) confirmed that the two mouse ALLs predicted to be PAX5 P80R had either Pax5 P80R homozygous mutations or a heterozygous mutation and a deletion affecting the remaining allele (Fig. 6b and Supplementary Data 8 and 9 ). Sanger sequencing confirmed these results and identified 6 of 53 (11.3%) ALLs with PAX5 P80R mutations (Supplementary Figs. 18 and 19 ). These findings highlight the relevance of our model for human B-ALL. Further, similar to humans, Ph-like mouse ALLs displayed mutations in genes involved in signal transduction, such as Kras [33] , as well as Flt3l, Limk1, Rem2 and Cdc42bpb (Fig. 6b and Supplementary Fig. 18 ). The latter two were also altered in one PAX5 P80R case. In addition, we found mutations in Trp53 , Kmt2d and FoxM1 (Fig. 6b and Supplementary Fig. 18 ), genes reported in human ALL [17] , [34] , [35] . Fig. 6: Mouse mutant IL7R leukemias resemble Ph-like and PAX5 P80R human B-ALL. a Principal component analysis (PCA) plot of gene expression profiles from mouse leukemia samples. b Mutational burden map of copy number variants (CNVs), single nucleotide variants (SNVs), and indel variants with predicted high and moderate impact in genes of interest. c Heatmap of PAM posterior probabilities classification of human Ph-like samples (from ref. [16] ) into the two apparent Ph-like subgroups observed in IL7R mutant leukemic mice. d Oncogenes and tumor suppressor genes significantly (adj. p < 0.05; moderate t -test) up- and downregulated, respectively, in leukemic samples as compared to controls. Log2 fold-changes (FC) are indicated for each gene. Source data are provided as a Source Data file. Full size image We noticed that PCA also segregated IL7R mutant-driven Ph-like ALLs into two transcriptionally distinct subsets (Fig. 6a ), which we named Ph-like 1 and 2. The top 1000 genes that separated Ph-like 1 from Ph-like 2 in PC1 showed enrichment for KEGG antifolate resistance and JAK–STAT signaling pathways, whereas those related to Ph-like 2 were enriched in, for instance, Wnt and Hippo signaling pathways (Supplementary Data 10 ). In agreement, Ph-like 1 displayed a stronger profile of activation of IL-7R downstream target genes than Ph-like 2 (Supplementary Fig. 20 ). In accord with higher IL-7R-mediated signaling in Ph-like 1, we found transcriptional enrichment in MYC and mTOR signaling in the Ph-like 1 subgroup versus Ph-like 2 (Supplementary Fig. 20 ). The two subgroups associated with different mutational patterns, with Ph-like 2 presenting mutations in regulators of chromatin remodeling and transcription ( Kmt2d , Suv39h1 , H3f3b and Hist1h3 ) and exocytosis/secretion ( Cadps2 ), that were absent from Ph-like 1 (Fig. 6b , Supplementary Fig. 21 and Supplementary Data 8 ). Conversely, Cdkn2a deletions, Kras mutations, and Gins2 gains were present exclusively in Ph-like 1 (Fig. 6b , Supplementary Fig. 21 and Supplementary Data 8 and 9 ). Gins2 was reported to promote survival and proliferation of K562 cells and there is an association between Gins2 expression levels and response to MTX in ALL [36] . Of note, these two IL-7R-related subsets are present in human ALL cases (Fig. 6c and Supplementary Data 11 ). Altogether, our data indicate that IL7R mutant-driven leukemias are either PAX5 P80R or Ph-like, in accord with these subtypes being enriched within mutant IL7R patients (Supplementary Data 12 ). Transcriptional alterations in oncogenes and tumor suppressors may also potentiate or collaborate with the effects of IL7R mutation. In addition to Myc and Bcl2 (Fig. 2i ), other tumor-promoting genes such as Eef2 and Myh10 were upregulated in leukemia cells, whereas tumor suppressors such as Ikzf1 , Ikzf2 , Arid1b , Arid2 , Samhd1 , Bach2 , and Myo18b were downregulated (Fig. 6d and Supplementary Data 4 ). Kras mutation cooperates with mutant IL7R To provide evidence that the gene lesions we identified cooperate with IL7R mutation in driving B-ALL, we next transduced IL7R mutant BM progenitors with Kras Q61H and transplanted them into lethally irradiated mice (Supplementary Fig. 22A ). IL7R mutant progenitors expressing Kras Q61H were able to reconstitute B cell development to a similar degree those transduce with empty vector or to IL7R wild-type progenitors expressing Kras Q61H (Supplementary Fig. 22B ). However, IL7R mutant Kras Q61H-expressing B cell precursors (GFP+) displayed larger size (indicative of increased metabolism and proliferation), higher surface levels of the IL-7R downstream target ENPEP/BP-1, and higher levels of IL-7R signaling target genes Cish , Asns , and Ccnd2 , as compared to control GFP-negative cells from the same transplants or empty vector-transduced cells (Supplementary Fig. 22C–E ). IL7R wild-type precursors transduced with Kras Q61H confirmed that these differences resulted mostly from the cooperation between mutant IL7R and mutant Kras , rather than from the effect of each oncogene alone (Supplementary Fig. 22C–E ). Importantly, one of seven transplanted IL7R mutant precursors transduced with Kras Q61H developed leukemia (Supplementary Fig. 23 ), whereas none of the controls showed any signs of leukemia development. These results indicate that Kras mutation cooperates with IL7R mutation in upregulating IL-7R-mediated signaling and accelerating leukemic transformation, suggesting that one of the possible mechanisms by which additional lesions cooperate with IL7R mutation in driving leukemia is the upregulation IL-7R-mediated signaling. Therapeutic targeting of IL7R mutant B-ALL We next explored our model to investigate ways to target therapeutically B-ALLs with IL-7R mutational activation. High PI3K/mTOR signaling pathway activation has been associated with disease aggressiveness and poor prognosis in B-ALL [37] , [38] . Because IL7R mutant leukemias exhibited clear upregulation of mTOR signaling, we administered the clinical-grade dual PI3K and mTOR inhibitor dactolisib (Fig. 7a ) and found it had a striking impact on the frequency of leukemia cells in the blood (Fig. 7b ), significantly prolonging the survival of transplanted mice (Fig. 7c ). This is consistent with observations in human Ph-like ALL patient-derived xenografts using another PI3K–mTOR inhibitor [39] . Fig. 7: Mutant IL7R B-ALLs are sensitive to PI3K/mTOR and SK pharmacological inhibition. a Dactolisib in vivo administration scheme. Leukemic cells (2 × 10 5 ) were transferred into Rag−/−γc−/− hosts. b Leukemia cell frequency detected in blood 6 days after treatment ( n = 10). Two-tailed, unpaired t -test. c Kaplan–Meier survival curves, and respective log-rank p value, of animals ( n = 7 control; n = 6 dactolisib) treated with vehicle or dactolisib (30 mg/kg). d Z -score values of chemical screen library for kinase inhibitors tested in IL-3-dependent Ba/F3 cells stably transduced with mutant IL7R and cultured in the absence of IL-3. Each compound is represented by one dot. SKi is denoted in red. Dotted lines represent Z -score cut-off. e Immunoblot analysis of STAT5 phosphorylation in Ba/F3 cells pre-treated with SKi (10 µM) or DMSO for 2 h and then stimulated with either IL-3 ( IL7R WT cells) or IL-7 ( IL7R mutant cells). IL7R WT-transduced cells were used merely as transduction controls for IL7R mutant cells but express IL-3R and respond to IL-3. IL-7 was used in IL7R mutant cells to reinforce IL-7R signaling while keeping the same period (30′) of cytokine stimulation as in IL-3-stimulated cells. This experiment was repeated once with identical results. f Viability, evaluated by FSC × SSC flow cytometry discrimination, of IL-3-cultured IL7R WT cells or IL-7-cultured IL7R mutant Ba/F3 cells treated with SKi or DMSO for 72 h. g Viability of leukemia cells from three independent mice, as compared to healthy B cell precursor controls in the presence of IL-7, cultured with increasing concentrations of SKi for 12 h. Viability index is normalized to the control condition (DMSO). Average ± s.e.m. is shown for each concentration. h Viability (Annexin V/7AAD expression) of representative leukemia cells incubated with SK2 inhibitor Compound 55 (20 µM) or DMSO for 12 h. i Dose-dependent effect of Compound 55 on leukemia cell viability ( n = 4; 2 PAX5 P80R and 2 Ph-like). j Compound 55 in vivo administration scheme. Leukemic cells (2 × 10 5 ) were transferred into Rag−/−γc−/− hosts. k Kaplan–Meier survival curves and respective log-rank p value of animals treated with vehicle ( n = 7) or Compound 55 ( n = 6; 5 mg/kg). l – n Viability of mutant IL7R human PAX5 P80R primary B-ALL cells cultured with increasing concentrations of ( l ) Dactolisib, ( m ) Compound 49, or ( n ) Compound 55 for 48 h. Viability index is normalized to the control condition (DMSO). Lines represent average of the duplicates, which are shown, for each patient sample. Source data are provided as a Source Data file. Full size image Next, to identify new targeted agents against mutant IL7R dependence, we performed a chemical screen using an 80-compound kinase inhibitor library on Ba/F3 cells ectopically expressing mutant IL-7Rα [13] . In addition to Cdk inhibitors, expected to counteract the effects of IL-7R-mediated signaling [40] , [41] , we found that a pan-sphingosine kinase (SK) inhibitor (SKi), which blocks the activity of both SK1 and SK2, efficiently prevented IL-7R-dependent cell growth (Fig. 7d and Supplementary Data 13 ). SK inactivation was not broadly cytotoxic, since the inhibitor abrogated only IL7R-, but not IL-3-, dependent signaling (Fig. 7e ) and viability (Fig. 7f ) of Ba/F3 cells. SKi also induced cell death in IL7R mutant mouse B-ALLs (Fig. 7g ). We validated this effect using new generation SK inhibitors [42] . Both the dual SK1/SK2 inhibitor Compound 49 and the isoform-specific SK2 inhibitor Compound 55 (ref. [42] ) promoted dose-dependent leukemia cell death in vitro (Fig. 7h, i and Supplementary Fig. 24 ), and were effective in vivo (Fig. 7j, k and Supplementary Fig. 24 ). Importantly, we validated our findings in human B-ALL. Similar to the mouse leukemia samples, pharmacological inhibition of PI3K and mTOR using dactolisib (Fig. 7l and Supplementary Fig. 25 ), or treatment with the SK inhibitors Compound 49 (Fig. 7m ) and Compound 55 (Fig. 7n ) had a clear inhibitory effect on two primary human diagnostic PAX5 P80R B-ALL samples presenting with IL7R type 1a gain-of-function mutations. The IL-7/IL-7R signaling axis has been implicated in T- and B-ALL. However, the lack of evidence that IL7R mutational activation per se could trigger leukemogenesis and the absence of models where mutation could be uncoupled from overexpression of the receptor prompted us to develop a conditional mutant IL7R knock-in mouse. A study parallel to ours, published while our manuscript was under revision, made use of a conditional floxed transgenic model where the IL7R mutation was introduced into the Rosa26 locus and expressed in B cell committed precursors, and demonstrated that mutant IL7R can drive B-ALL [43] . However, the strategy used leads to the expression of the mutant receptor downstream of an ubiquitously expressed promoter, implicating that the mutant IL7R is not physiologically regulated (hence it will be either over- or ectopically expressed throughout B cell development) and is aberrantly expressed in the context of two wild-type IL7R alleles. This is of particular relevance, as we recently demonstrated that overexpression of the wild-type IL7R can be oncogenic [44] . In contrast, in our model, mutant IL7R expression is kept under physiological regulation—similar to what happens in human ALL, where no mutations in promoter, enhancer, or super-enhancer regions directly regulating IL7R have been reported. Our results demonstrate that IL7R gain-of-function mutation initiates leukemia by causing a pre-leukemic stage in B cell precursors with evidence of self-renewal activity. Our findings are coincident with those in human hematopoietic precursor cells, arising from parallel studies conducted by Geron et al., demonstrating the ability of mutant IL7R to induce a pre-leukemic stage with self-renewal ability ( https://doi.org/10.1101/2020.01.27.919951 ). We further show that pre-leukemia cells display higher viability, but not proliferation, than healthy B cell precursors and eventually transform, likely by the accumulation of mutations (e.g. Kras Q61H) that tend to contribute to increased IL-7R-mediated signaling and proliferation, into full-blown leukemia with characteristics of PAX5 P80R or Ph-like ALL. These are precisely the subsets where IL7R mutations are most frequent in humans [16] , [17] . The relatively long median latency for leukemia development in the IL7R mutant heterozygous mice is also consistent with the fact that Ph-like ALL is predominant in older patients. Although IL7R mutations are frequently subclonal in human ALL, indicating they occur late in leukemia development, there are cases of Ph-like B-ALL where IL7R mutant allele frequency is compatible with IL7R mutation being the initiating lesion [16] , [45] . Likewise, although PAX5 P80R mutations are known to be the initiating event in this ALL subtype [16] , IL7R and PAX5 mutant allele frequencies are, in some cases, compatible with the possibility of IL7R mutation initiating the disease with subsequent early acquisition of PAX5 mutations [16] . In agreement, PAX5 P80R lesions occur in our IL-7R-driven model (in around 11% of the cases), suggesting a strong selective advantage in the combination of IL7R and PAX5 mutations. Mutations and copy number alterations in genes affected in human B-ALL included also Trp53 , FoxM1 , Cdkn2a , Kras , and Kmt2d , underlining the relevance of our model to dissect the etiology of this malignancy. Moreover, lesions affecting these genes cooperate with IL7R mutation, likely contributing to increased proliferation, as shown by our studies with mutant Kras and consequent upregulation of Ccnd2 , and those of Geron et al., which showed deletion of CDKN2A in a B-ALL arising from the in vivo transplantation of human cord blood progenitors transduced with mutant IL7R and demonstrated cooperation between IL7R mutation and CDKN2A deletion in driving human B-ALL ( https://doi.org/10.1101/2020.01.27.919951 ). Also noteworthy are the two IL7R-triggered Ph-like ALL transcriptional subgroups, one of which (Ph-like 1) displays Cdkn2a deletions, Kras mutations and Gins2 gains and the other (Ph-like 2) mutations in genes encoding histone methyltransferases ( Kmt2d , Suv39h1 ) and histone subunits ( H3f3b and Hist1h3 ). Although kinase and signaling-related gene alterations, such as those affecting Ras , are a hallmark of human Ph-like ALL [46] , mutations in histones and chromatin regulators can also occur in this subset [17] , [47] . Notably, we found transcriptional counterparts to both mouse Ph-like subsets in human leukemia. Nonetheless, the two Ph-like transcriptional subsets we identified and their respective mutational characteristics need further validation in a larger number of animals and, especially, in the human setting. In our model, IL7R mutational activation occurred from the CLP stage onwards. However, we did not detect any major alterations in T cell development or the occurrence of T cell ALL, despite obvious expression of the mutant IL7R in the T cell lineage. In T cells, IL-7R-mediated signaling leads to IL7R transcriptional downregulation [48] , and IL-7 stimulation decreases IL-7Rα surface expression due to increased trafficking to the early endosome and subsequent degradation [49] . These constitute obstacles to excessive signaling in T cells not shared by B cell precursors, which may help explain the skew towards B-ALL that we observed. The limits to IL-7R-mediated transformation in B- versus T-cell precursors warrant further investigation. Leukemia development occurs in a majority of heterozygous, and in all homozygous, Il7r mutant mice, contrasting with previous studies showing that STAT5 activation alone leads to B-ALL with very low penetrance and long latency [50] . This indicates that IL-7R-mediated leukemogenic effects extend beyond those of the JAK–STAT pathway, in line with the knowledge that IL-7R triggers other oncogenic signaling pathways [7] . In fact, we showed that IL7R mutant ALL cells rely not only on JAK and STAT5, but also on PI3K–mTOR activity. These observations suggest that the combination of distinct survival and proliferative pathways (e.g. JAK–STAT and PI3K–mTOR) triggered by mutant IL7R likely compensates for possible barriers to transformation imposed to the activation of each pathway separately [51] , overall resulting in strong oncogenic potential. The ability of high IL-7R-mediated signaling levels to drive ALL is illustrated in mutant IL7R homozygous mice, whose B cell precursors undergo transformation in a very rapid and polyclonal fashion (indicating a strong ability to transform), and with less moderate/high impact mutations (indicating higher signaling requires less cooperating hits to drive leukemia). The results from IL7R homozygous mice would also be compatible with wild-type IL-7R acting as a tumor suppressor. However, this is unlikely, since most evidence in T- and B-ALL suggests that high IL-7R wild-type signaling is oncogenic [11] , [25] , [44] , [52] . While increased signaling in homozygous versus heterozygous IL7R mutant leukemias may potentially result from increased expression of the mutant form and/or absence of the wild-type IL7R, the end-result is markedly increased signaling and increased oncogenic potential. We identified transcriptional and mutational alterations that may contribute to leukemogenesis downstream from IL7R mutation. IL-7R-dependent Myc upregulation is an obvious candidate, especially taking into account that survival effectors (such as Bcl-2) activated by mutant IL-7R-mediated signaling will likely counterbalance possible pro-apoptotic effects of Myc activation [53] . MYH10 encodes non-muscle myosin heavy chain IIb, and is upregulated in different cancers, including myeloid leukemias [54] . Myh10 was upregulated in IL7R mutant leukemias. Curiously, other regulators of motility were also affected in the leukemic samples, namely the tumor suppressor Myo18b [55] that was downregulated, and Cdc42bpb (encoding Mrckb) and Limk1 (known to be phosphorylated by Mrckb) that were mutated. Altogether, this suggests that IL-7R signaling can activate and/or cooperate with a program involved in tumor spreading. Whereas we did not find mutations in tumor suppressors such as Arid1b , which is mutated in human B-ALL [17] , there was clear transcriptional downregulation that extended to Arid2 . Similarly, we did not detect genetic alterations in Ikzf1 (encoding Ikaros), and found only mild downregulation in Ikzf1 transcript levels. Although IKZF1 deletions are a hallmark of Ph-like ALL [15] , [56] , they in fact tend not to co-segregate with IL7R mutations within this subset. Only 20% of exon 6 IL7R indel mutant cases display IKZF1 alterations, whereas samples with ABL-class fusions (71%), CRLF2 rearrangements (77%), and EPOR or JAK2 rearrangements (86%) show considerably higher frequencies [15] . Mechanistically this is not surprising, since Ikaros competes with IL-7R-dependent signaling in B cell development and is displaced by STAT5 during leukemogenesis [50] , [57] . This implies that high signaling levels from mutant IL-7Rα will tend to render Ikaros functionally obsolete without the need for mutational inactivation. Comparison of drug sensitivity of mutant IL7R human B-ALL samples with B-ALLs arising in our mouse model validated its use in the search for novel therapeutic avenues. Previous studies showed that BET bromodomain [32] or JAK [58] inhibitors can target IL-7R-related high risk ALL. Here, we demonstrated that PI3K-mTOR inhibition is an additional strategy—of particular relevance given the association of mTOR activation with poor prognosis in B-ALL [37] , [38] . Moreover, in the sequence of our kinase-directed functional screening, we demonstrated that SK pharmacological inhibitors abrogate IL-7R-mediated signaling, promote mutant IL7R ALL cell death, and delay tumor growth. This is in line with the knowledge that SK activity promotes B-ALL [59] , and indicates that SK small-molecule inhibitors may be particularly useful against IL-7R-dependent B-ALL cases. In summary, we generated an in vivo model that formally demonstrates that IL7R gain-of-function drives bona fide precursor B-ALL and, importantly, can initiate the disease. Our model constitutes a resource to characterize new molecular and cellular players in B-ALL etiology, in the context of otherwise normal hematopoietic development, and to test new therapeutic approaches in an immunocompetent setting. Mouse models All animal experiments were performed according to the regulations of Instituto de Medicina Molecular João Lobo Antunes (IMM-JLA) and Portuguese and European legislation. Il7r flCPT conditional knock-in animals in C57Bl/6 background were generated by Cyagen Biosciences (Santa Clara, CA). Il7r exon 6 was targeted by a homologous recombination vector carrying the wild-type exon 6 and a reversely positioned mutant exon 6 in conjunction with a Neomycin (Neo) selection cassette and flanking 5′ and 3′ homology arms. The mutant exon 6 consisted of an in-frame insertion of TGTCCCACC, coding for cysteine (C), proline (P), and threonine (T), at the coding sequence nucleotide position 733 (Supplementary Fig. 1A ). The Neo cassette, flanked by Frt sites, was deleted from the conditional knock-in (KI) allele by crossing the transgenic mice with a strain expressing the yeast Flp recombinase. 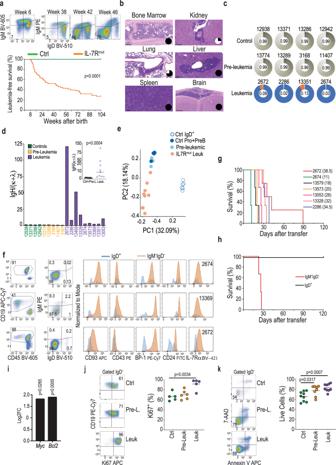Fig. 2: IL-7Rα mutant mice develop precursor B-ALL. aExample of IgM−IgD−cell frequency evolution in a mouse that developed leukemia (top). Kaplan–Meier leukemia-free survival curves of control (Ctrl;n= 40) andIL7Rmutant (IL7Rmut;n= 63) animals (bottom). All mice died with precursor B-ALL. Log-rank Mantel–Cox test (b) Histologies (H&E) of organs infiltrated with leukemia cells. Pie chart inserts represent fraction of analyzed animals (n= 4) with leukemia involvement (in black) in the respective organ. Scale bar indicates 100 μm (bone marrow, spleen), 250 μm (kidney, lung, liver), or 500 μm (brain).cClonality pie charts based onIgHsequencing. Each colored slice corresponds to a clone, indicative of clonality. Gray areas correspond to many rare clones, indicative of polyclonality. Equitability values (ranging from 0, for monoclonality, to 1, for a balanced repertoire) are shown in the center of the pie charts. Samples are bone marrow pro+pre-B cells from control, pre-leukemic, or leukemic mice.dIg heavy chain (H) over light chain (κ and λ) ratios to evaluate, at the population level, the presence of the pro-B cell rearrangement signature (heavy chain expression in the absence of light chain expression). Two-tailed Mann–Whitney test performed.ePrincipal component analysis of normal (Ctrl Pro+Pre-B) and pre-leukemic (Pre-leukemic) pro- and pre-B cell precursors, mature splenic B cells (Ctrl IgD+) and leukemia cells (IL7RmutLeuk).fImmunophenotypic analysis of three representative BM leukemia samples. Numbers inside dot plots indicate frequency in each quadrant or region.g,hKaplan–Meier leukemia-free survival curves of mice transplanted withgbulk primary leukemias orhsorted IgD+versus IgM−IgD−leukemia cells.iMycandBcl2transcript upregulation (log2 fold change) in leukemia samples (n= 9) as compared to normal controls (n= 5). Moderatedt-test performed.jFrequency of Ki67-positive cells in controls (n= 5), pre-leukemia (n= 5), and leukemia samples (n= 5). Dot plots are representative of each condition.kFrequency of annexin V/7AAD-negative (viable) cells in controls (n= 9) pre-leukemia (n= 8) and leukemia samples (n= 9). Dot plots are representative of each condition.j,kTwo-tailed unpairedt-test. Source data are provided as a Source Data file. Supplementary Figure 2A shows the conditional knock-in allele after Neo deletion. Exon 6 and mutant exon 6 were flanked by LoxP and Lox511 sequences in a FLEX switch configuration [60] , [61] . The LoxP and the variant Lox511 sites were arranged in such a configuration (place, distance, and orientation) that, upon Cre recombinase activity, the mutant and wild-type exons 6 are inverted, positioning the mutant exon 6 in the sense orientation and deleting the wild-type exon 6 (Supplementary Fig. 2A ). In keeping with the guidelines set by the International Committee on Standardized Genetic Nomenclature for Mice, our KI mouse strain was named C57BL/6J-Il7r <tm1(CPT)> or B6-Il7rtm1(CPT) where “(CPT)” accounts for the CysProThr insertional-mutation. Hereafter, it will be referred to as Il7r flCPT (fl = floxed). Genotyping of the Il7r flCPT allele was carried out with primers F1 and R1 (all primer sequences can be found in Supplementary Data 17 ). Heterozygous mutant mice were identified through the presence of a 352 bp fragment from the wild-type allele and of a 521 bp fragment resulting from the recombinant allele. To confirm the Cre-mediated recombination of the floxed Il7r flCPT allele, primer F1 and F2 were used. This results in a 1067 bp band from the loxP/Lox511 inverted/excised allele. hCD2-iCre, B6 Rag −/− γc − /− and NSG animals were bred and kept at the IMM-JLA SPF animal facility. In all experiments, animals were closely monitored and sacrificed when reaching humane endpoints: loss of 20% of body weight, hind leg paralysis, breathing impairment, or poor reaction to external stimuli. Experiments were performed according to the IMM-JLA’s institutional (including ORBEA Ethical Review approval) and Portuguese (DGAV) regulations. Animals were kept in ventilated systems at 20–24 °C, and relative humidity of 55 ± 10%, with controlled supply of High Efficiency-Particulate Air (HEPA) filtered air provided to individually ventilated cages. 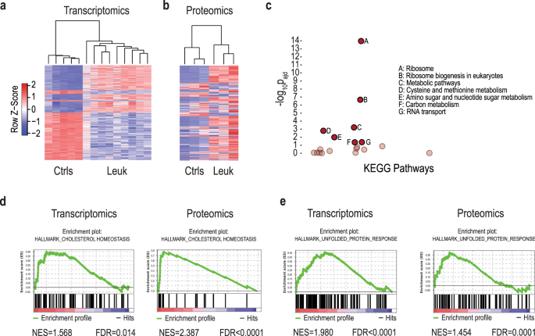Fig. 3: Transcriptomics and proteomics characterization of mutantIL7Rleukemias. aHeatmap representation and hierarchical clustering of control and leukemia samples based on the 1000 most significant (adj.pvalue) differentially expressed genes.bHeatmap representation of samples based on the 500 most significant (nominalpvalue) differentially expressed proteins between control and leukemia samples.cg:Profiler KEGG pathway functional enrichment analysis for significant and concordantly upregulated genes and proteins in leukemia samples. Significantly enriched pathways (A–G, adj.p< 0.05. Cumulative hypergeometric test) are represented in full opacity. Pathways below the significance threshold are represented in low opacity. Pathways wherep= 1 are not featured.d,eGene set enrichment analysis (GSEA)-enrichment plot of differential gene and protein expression between leukemias and controls showing a significant upregulation of thedcholesterol homeostasis and theeunfolded protein response (UPR) hallmark gene sets (normalized enrichment score (NES) > 1, FDR < 0.05). Source data are provided as a Source Data file. Maximum number of animals per cage was 5. Social isolation was avoided whenever possible. Rooms’ light/dark cycle was 14 h Light:10 h Dark. Type of food was autoclaved diet pellets RM3A (P), from SDS Special Diets Services (Product code: 801030). Food was placed in a grid inside the cage and provided ad libitum to animals. Leukemia incidence A cohort of experimental animals was weekly weighed and bled, and sacrificed in a CO 2 chamber or via pentobarbital injection when reaching humane endpoints. In addition to the BM, disseminated disease was confirmed by collecting thymus, spleen, and liver samples for flow cytometry and histological analysis. Experiments were terminated at 104 weeks of age. Differences in survival curves were determined by Log-rank (Mantel–Cox) test using Prism v8.0. Leukemic cell transfer 2 × 10 5 sorted leukemic cells were transferred i.v. via the tail vein into sex- and age-matched 8–20-week-old hosts. Animals were monitored daily, weighed, and bled for immunophenotyping weekly and sacrificed in a CO 2 chamber or via pentobarbital injection when reaching humane endpoints. In the absence of disease, experiments were terminated 120 days after transfer. Self-renewal experiments 8–10-week-old sex-matched hosts were sub-lethally irradiated (350 rad) and transferred with 2 × 10 6 sorted pro+pre-B cells from control or IL-7R mut animals in first transfer and 10 7 total BM cells in secondary transfers. Animals were monitored daily, weighed weekly, and sacrificed in a CO 2 chamber or via pentobarbital injection when reaching humane endpoints. In vivo Ba/F3 tumor growth Ba/F3 cells expressing the murine wild type or mutant Il7r were injected subcutaneously into the right and the left flank (respectively) of 11-week-old NSG mice (5 × 10 6 cells in 100 μl of PBS). Mice were monitored for tumor development and tumor size measured by a caliper. Tumor volume was calculated using the formula: tumor volume = ½ (length × width 2 ). Mice were euthanized when tumors reached a volume of 1000 mm 3 . In vivo treatment of leukemia Sorted leukemia cells (2 × 10 5 ) were transferred into Rag −/− γc −/− hosts and animals were monitored daily and minimally bled (<20 µL) for FACS determination of leukemia cells (CD19 + ) at days 7 and 10 after transfer. Upon leukemia detection in all animals (mCD45 + CD19 + > 0.5%), mice were randomized into treated and control groups. The PI3K/mTOR inhibitor Dactolisib (BEZ235, NVP-BEZ235; Selleckchem)—dissolved v/v 10 NMP and 90 PEG300 (Sigma Aldrich)—was administered daily at 30 mg/kg by oral gavage for 15 days, whereas vehicle was administered to the control group. 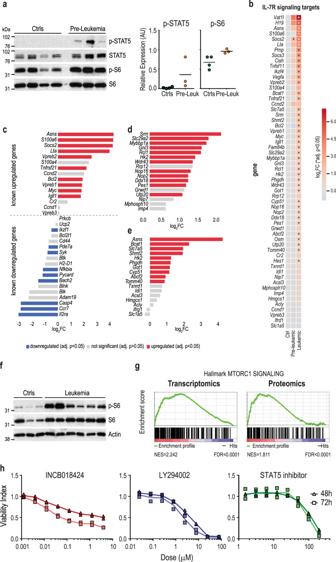Fig. 4: Leukemia cells rely on IL-7R signaling, which boosts upon transformation. aImmunoblot analysis of phosphorylated STAT5 and S6 levels in sorted pro+pre-B cells from control (n= 4) and pre-leukemic (n= 3) mice, IL-7-deprived for 12 h. Graphs represent densitometry values for P-STAT5 and P-S6 normalized to respective total protein.bDifferential gene expression of known IL-7R signaling targets in pre-leukemia and leukemia samples compared to controls (reference category). Moderatet-test performed.c–eDifferential expression of (c) STAT5, (d) MYC, and (e) mTOR targets in leukemia versus control samples. Significantly upregulated and downregulated genes (adj.p< 0.05; moderatet-test) are shown in red and in blue, respectively.fImmunoblot analysis of phosphorylated S6 levels in control (n= 3) and leukemia (n= 6) samples analyzed ex vivo.gTranscriptomic and proteomic gene set enrichment analysis (GSEA) showing a significant enrichment of the mTOR signaling hallmark gene set in leukemias versus controls.hLeukemia cells were cultured in the presence or absence of pharmacological inhibitors of JAK1/2 (INCB018424; ruxolitinib), STAT5 (STAT5 inhibitor), and PI3K (LY294002) at the indicated doses, and viability was evaluated at 48 and 72 h. Results from a representative mouse (n= 3). Lines represent average of duplicates that are shown. Source data are provided as a Source Data file. Treatment was then stopped for 12 days and subsequently restarted for 13 days. Animals were sacrificed when reaching humane endpoints. Animals without disease symptoms were sacrificed 120 days after cell transfer. For sphingosine kinase inhibitor treatment, sorted leukemia cells (2 × 10 5 ) were transferred into Rag −/− γc −/− hosts and 1 day after injection animals were randomized into three groups: compound 49, compound 55, or vehicle (20% cyclodextrin/PBS). Both compounds were administered daily at 5 mg/kg by intraperitoneal injection for 21 days. Animals were monitored daily and bled weekly for FACS detection of leukemia cells (CD19 + ). Animals were sacrificed when humane endpoint was reached. Differences in survival curves were determined by log-rank (Mantel–Cox) test using Prism v8.0. Histopathology Samples were immersion-fixed in 10% neutral buffered formalin, routinely processed for paraffin embedding, sectioned at 4 µm, stained with hematoxylin and eosin, and examined by a pathologist blinded to experimental groups. Tumor cell infiltration was scored according to a 5-tier severity scale: 0, absent; 1, minimal; 2, mild; 3, moderate; 4, marked, and representative photographs were acquired using NDP.view2 software (Hamamatsu) in slides digitally scanned in the Hamamatsu NanoZoomerSQ. Immunophenotyping Blood was collected into tubes with heparin and red blood cells (RBCs) were lysed with lysis solution (Becton Dickinson San Jose, CA, USA), prior to staining with standard procedures. Splenic, thymic and BM single-cell suspensions were immunophenotyped using standard methodology. Briefly, 10 6 cells were stained for 20 min at 4 °C in PBS with 2% FBS with specific antibodies (Supplementary Data 14 ). 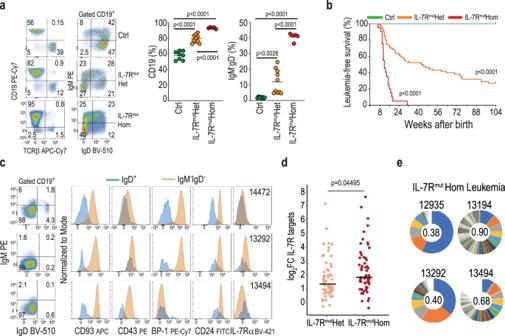Fig. 5: Homozygous expression of mutant IL7R leads to maximal IL-7R signaling hyperactivation and rapidly fatal leukemia. aDot plots of CD19 by TCRβ to identify T and B cell lymphocytes in blood at 6 weeks of age in representative animals of indicated genotypes (left) and graphs summarizing data from all animals analyzed (right). Ctrls:n= 8; IL-7RmutHet:n= 10; IL-7RmutHom:n= 5. Each dot denotes an animal and mean value is shown. Numbers in dot plots indicate frequency in each quadrant. One-way ANOVA.bKaplan–Meier leukemia-free survival curves of control (n= 40), IL-7RmutHet (n= 63), and IL-7RmutHom (n= 20) mutant animals. Log-rank (Mantel–Cox) test. All mice died with precursor B-ALL.cImmunophenotypic analysis of three representative BM IL-7RmutHom leukemia samples. Numbers inside dot plots indicate frequency in each quadrant or region.dComparison of IL-7R “signaling strength” between IL-7RmutHet and IL-7RmutHom leukemia samples, as measured by the levels of differential gene expression over control samples. Each dot represents log2 fold change (FC) of an IL-7R signaling target gene (see Fig.4b). Means are indicated. Unpaired two-tailedt-test.eClonality pie charts based onIgHsequencing (see Fig.2cfor further details). Source data are provided as a Source Data file. When lineage-positive cells were excluded, biotin coupled anti-Gr-1, CD11b, CD19, Ter119, NK1.1, and CD11c were used and subsequently stained with BV711 streptavidin. Proliferation was analyzed by intracellular staining of Ki67 (APC-conjugated, Biolegend), using the Foxp3 staining kit from eBioscience and following the manufacturer’s instructions. Cell viability was determined using an annexin V-based apoptosis detection kit and following the manufacturer’s instructions (eBioscience). 10-color analyses were performed on LSR Fortessa II (Becton Dickinson San Jose, CA, USA) flow cytometers. Results were analyzed with FlowJo (Tree StarInc., Ashland, OR, USA) software. Gating strategies used are exemplified in Supplementary Figs. 26 – 30 . FACS cell sorting BM and spleen cell suspensions were stained for sorting with anti-CD19, B220, IgM, IgD, CD45, and TCRβ and sorted on a FACSAriaIII (Becton Dickinson San Jose, CA, USA). Leukemia cells were sorted from BM or spleen samples as CD45 +or − CD19 + IgM − IgD − ; pro+pre-B precursors were sorted from the BM as CD45 int B220 int IgM − ; mature B cells were sorted from the spleen as CD45 + CD19 + IgD + ; and T cells as CD45 + TCRβ + . Retrovirally transduced cells were stained and sorted as CD19 + GFP + or CD19 + GFP − , 3 days after transduction. Cells were then resuspended in IMDM for further culture or in PBS for transfer into recipient animals. WES and data analysis DNA from sorted cells was extracted with Qiagen ALLprep extraction kit. Sequencing was performed as previously detailed [16] . WES data processing and variant calling were performed by RubioSeq software v3.8a ( http://rubioseq.bioinfo.cnio.es/ ) using default parameters for somatic variation analysis [62] . Briefly, sequencing data were first checked by FastQC for quality control on raw sequence data and then aligned to the mouse reference genome (mm10) using Burrows-Wheeler alignment (BWA) [63] . Reads unmapped by BWA were realigned using BFAST [64] . For variant calling we used GATK Unified Genotyper v2 (ref. [65] ), applying the “Discovery” genotyping mode and default parameters for filtering. The GATK QUAL field was employed for ranking selected somatic variants. Variants were annotated with SnpEff 4.3r (VEP) [66] . Variants were filtered to ensure that each variant had at least a coverage over 30. Additional filters were applied for the specific identification of somatic variants; loci showing high numbers of variants exclusively present in sibling mice were not considered, and variants present in the Mouse Genome Project [67] most recent release (v6) for SNPs and indels were also filtered out. For somatic copy number variation calling, the aligned WES bam files of leukemic and control mouse models as well as the corresponding bed file indicating exon target positions were used for somatic copy number variation (CNV) calling using the CODEX2 pipeline [68] . As a case–control design, CNVs disproportionately present in the leukemic mouse models compared to the controls were detected. In brief, GC content and mappability for each exon region was calculated from the mm10 reference genome. Depth of coverage matrices for each chromosome was built and sample- and exon-wise quality control regarding coverage, length, mappability, and GC content, was performed using default settings, before subjected to the CODEX2 algorithm background estimation, normalization, and CNV detection based on poisson-likelihood based recursive segmentation [69] . The fractional mode was used as the objective is to call somatic variant. The CNV events were categorized and number-coded to be amplification (+2), gain (+1), diploid (0), heterozygous deletion (−1), and homozygous deletion (−2), for cases where the estimated exact copy number ratio was >3.3, 2.3–3.3, 1.7–2.3, 0.7–1.7, and <0.7, respectively, as previously described [68] . The categorical CNV events were then visualized and examined using the Integrative Genomics Viewer version 2.4.16 (ref. [70] ). Waterfall plot for variants was generated using R (v3.4.4, https://www.R-project.org/ ) and the GenVisR package (v1.8.1). RNA sequencing (RNA-seq) and data analysis RNA was extracted from sorted cells with Qiagen ALLprep extraction kit. Sequencing was performed as previously described [16] . RNA-seq data quality was assessed using FASTQC (v0.11.7, https://www.bioinformatics.babraham.ac.uk/projects/fastqc/ ). Reads were pseudo-aligned to mouse transcriptome (gencode M14) with Kallisto v0.44.0 [71] . Differential expression was assessed using edgeR (v3.20.9) and limma (v3.34.9) R packages [72] , [73] . Briefly, samples comparison was performed using voom transformed values, linear modeling and moderated T -test as implemented in limma R package, selecting significantly differentially expressed genes with FDR adjusted P values lower than 0.05. IL7R allele-specific expression levels were obtained using samtools [74] and bedtools [75] , converting to allele proportions for reference (wild-type) and mutant IL7R alleles. Principal component analysis (PCA) was performed using the stats package (v3.4.4) on voom transformed expression values. PCA plots were generated using the ggfortify (v0.4.8) and ggplot2 (v3.2.1) packages in R. Heatmap of transcriptional differences was generated with R package gplots with clustering performed with hclust from the R stats package. IL-7R, STAT5, Myc, and mTOR signaling targets were curated from the literature, differential expression heatmaps were generated with the seaborn (v0.9.0) and matplolib (v3.1.0) packages in Python 3.7.3, barplots were generated with ggplot2. We used MixCR framework to quantify clonotypes from transcriptome profiles using the recommended protocol for RNA-Seq [76] . Classification of IL-7R mutant mouse tumors was performed using human B-ALL transcriptome profiles [16] and nearest shrunken centroids as implemented in pamR (v1.56.1) R package ( https://cran.r-project.org/web/packages/pamr/index.html ). Briefly, human-mouse orthologs were first obtained from Ensembl v95 through “biomaRt” R package [77] . Second, human and mouse transcriptome profiles were quantile normalized using preprocessCore (v1.40.0) R package ( https://github.com/bmbolstad/preprocessCore ). Third, the human transcriptome data were split in two sets enclosing seven human B-ALL subtypes known to display (PAX5 P80R, IKZF1 N159Y, iAMP21, Ph-like) or not (DUX4, ETV6-RUNX1, and KMT2A) IL7R mutations: approximately 74% of samples within each subtype were used to train the classifier and 26% to evaluate its prediction capability. Finally, the classifier was used to assign the IL7R mutant mouse tumors according to the human B-ALL subtypes. The pamR packaged was also used to assess the distribution of human Ph-like B-ALL samples [16] among the seemingly two subgroups of Ph-like mice leukemias identified, where all mice from both subgroups were utilized for training of the classifier. Sanger sequencing Genomic DNA from sorted leukemia cells was extracted using AllPrep® DNA/RNA/Protein kit (Qiagen) following the manufacturer’s instructions. PCR was performed with 50 ng of genomic DNA using either Taq DNA Polymerase (Thermo Scientific) or Recombinant Taq DNA Polymerase TaKaRa Taq™ (Takara Bio) using the primers listed in Supplementary Data 15 . Sanger sequencing was performed using GATC services. Quantitative real-time PCR RNA was retro-transcribed using High Capacity RNA-to-cDNA Kit, followed by a pre-amplification PCR using TaqMan PreAmp Master Mix. TaqMan Gene Expression Master Mix was used in real-time quantitative PCR performed in a 7500fast or ViiA7 real-time system (all from Applied Biosystems). TaqMan Gene Expression Assay (Applied Biosystems) was Hprt1 (Assay ID: Mm00446968_m1), Asns (Assay ID: Mm00803785_m1), Ccnd2 (Assay ID: Mm00438070_m1), and Cish (Assay ID: Mm01230623_g1). Expression of the mutated form of Il7r was detected in cDNA obtained from leukemic samples by RT-PCR analysis using custom Taqman probes and Gene Expression Master Mix. Expression of the mutant form of Kras (Q61H) was detected in retrovirally transduced cells, as described above, using Syber Green dye according to the manufacturer’s instructions. Gene expression analysis from RT-PCR analysis was calculated with the comparative CT method 2 −ΔΔCT . FASP processing of samples for proteomics Cell pellets were solubilized in Tris-HCl (100 mM, pH 8) containing 4% SDS and 100 mM DTT. Cell lysates were heated at 95 °C, and DNA was shredded by sonication. Samples were processed using FASP protocol [78] with some modifications. After, lysates were passed through filters (Nanosep, 10k, PALL Life Sciences), proteins were alkylated in 100 µL iodoacetamide at a final concentration of 50 mM for 15 min, filters were washed three times with 200 µL 8 M urea in Tris-HCl (100 mM, pH 8) then twice with 200 µL 40 mM ammonium bicarbonate. Proteins on the filters were then digested twice at 30 °C with trypsin (3.3 µg ×2), first overnight and then for another 6 h in 200 µL, ammonium bicarbonate at 40 mM. Resulting tryptic peptides were desalted using C18 solid phase extraction cartridge (Empore, Agilent technologies). LC-MS analysis for proteomics Analysis of peptides was performed on a Q-exactive-HF-X (Thermo Scientific) mass spectrometer coupled with a Dionex Ultimate 3000 RS (Thermo Scientific). LC buffers were the following: buffer A (0.1% formic acid in Milli-Q water (v/v)) and buffer B (80% acetonitrile and 0.08% formic acid in Milli-Q water (v/v). Aliquots of 5 μL of each sample were loaded at 10 μL/min onto a trap column (100 μm × 2 cm, PepMap nanoViper C18 column, 5μm, 100 Å, Thermo Scientific) equilibrated in 2% buffer B. The trap column was washed for 4 min at the same flow rate and then the trap column was switched in-line with a Thermo Scientific, resolving C18 column. The peptides were eluted from the column at a constant flow rate of 300 nL/min with a linear gradient from 5% buffer B to 35% buffer B in 116 min, and then to 98% buffer B by 118 min. The column was then washed with 98% buffer B for 15 min and re-equilibrated in 2% buffer B for 31 min. Q-exactive HF-X was used in data-dependent mode. A scan cycle comprised MS1 scan ( m / z range from 335 to 1800, with a maximum ion injection time of 50 ms, a resolution of 60,000 and automatic gain control (AGC) value of 3 × 10 6 ) followed by 40 sequential dependent MS2 scans (with an isolation window set to 1.4 Da, resolution at 7500, maximum ion injection time at 50 ms and AGC 10 5 , stepped collision energy was set to 27, and fixed first mass to 120 m / z . Spectrum was acquired in centroid mode and all unassigned charge states as well as singly charged species were rejected. To ensure mass accuracy, the mass spectrometer was calibrated on the first day that the runs were performed. Proteomics data analysis Raw mass spec data files were searched using the MaxQuant software package (version 1.6.0.1). Proteins and peptides were identified using a Uniprot canonical plus isoforms database (accessed 02/08/2017). The following search parameters within MaxQuant were selected: protein N-terminal acetylation and methionine oxidation were set as variable modifications and carbamidomethylation of cysteine residues was selected as a fixed modification; trypsin selected as digestion enzyme with up to two missed cleavages; the false discovery rate was set at 1% for protein and peptide and the match between runs function was disabled. Proteins were removed from the data set which were categorized as “reverse”, “contaminant” or “only identified by site”. Estimates of protein copy numbers per cell were calculated using the histone ruler method [79] within the Perseus package [80] . Differential protein expression was performed using the DEP (version 1.0.1) and limma (v3.34.9) packages in R (v3.4.4). Molecules showing nominal p < 0.05 were considered significant. Pathway enrichment analysis Two approaches were used to perform pathway enrichment analysis. Gene set enrichment analysis (GSEA) was performed on transcriptomic and proteomic data with GSEA v.4.0.3 (ref. [81] ), using the GSEAPreranked method with limma moderate t-statistic values as the gene ranking statistic against Molecular Signature Database (MsigDB)’s hallmark gene sets [82] using 1000 permutations with a specific seed for reproducibility. Pathways with a false discovery rate (FDR) < 0.05 were considered significant. Additionally, a more integrative approach was taken by identifying concordantly significantly differentially expressed genes (adj. p < 0.05) and proteins (nominal p < 0.05) between IL-7R mut het and controls. Genes in these conditions were queried in g:profiler’s g:GOSt functional profiling tool against Kyoto Encyclopedia of Genes and Genomes (KEGG) pathways. Significance was set at adj. p < 0.05 using the tool’s suggested g:SCS multiple comparison correction method. 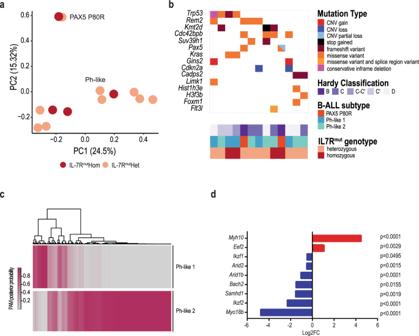Fig. 6: Mouse mutantIL7Rleukemias resemble Ph-like and PAX5 P80R human B-ALL. aPrincipal component analysis (PCA) plot of gene expression profiles from mouse leukemia samples.bMutational burden map of copy number variants (CNVs), single nucleotide variants (SNVs), and indel variants with predicted high and moderate impact in genes of interest.cHeatmap of PAM posterior probabilities classification of human Ph-like samples (from ref.16) into the two apparent Ph-like subgroups observed inIL7Rmutant leukemic mice.dOncogenes and tumor suppressor genes significantly (adj.p< 0.05; moderatet-test) up- and downregulated, respectively, in leukemic samples as compared to controls. Log2 fold-changes (FC) are indicated for each gene. Source data are provided as a Source Data file. 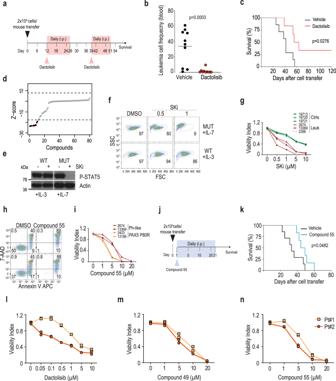Fig. 7: MutantIL7RB-ALLs are sensitive to PI3K/mTOR and SK pharmacological inhibition. aDactolisib in vivo administration scheme. Leukemic cells (2 × 105) were transferred into Rag−/−γc−/− hosts.bLeukemia cell frequency detected in blood 6 days after treatment (n= 10). Two-tailed, unpairedt-test.cKaplan–Meier survival curves, and respective log-rankpvalue, of animals (n= 7 control;n= 6 dactolisib) treated with vehicle or dactolisib (30 mg/kg).dZ-score values of chemical screen library for kinase inhibitors tested in IL-3-dependent Ba/F3 cells stably transduced with mutantIL7Rand cultured in the absence of IL-3. Each compound is represented by one dot. SKi is denoted in red. Dotted lines representZ-score cut-off.eImmunoblot analysis of STAT5 phosphorylation in Ba/F3 cells pre-treated with SKi (10 µM) or DMSO for 2 h and then stimulated with either IL-3 (IL7RWT cells) or IL-7 (IL7Rmutant cells).IL7RWT-transduced cells were used merely as transduction controls forIL7Rmutant cells but express IL-3R and respond to IL-3. IL-7 was used in IL7R mutant cells to reinforce IL-7R signaling while keeping the same period (30′) of cytokine stimulation as in IL-3-stimulated cells. This experiment was repeated once with identical results.fViability, evaluated by FSC × SSC flow cytometry discrimination, of IL-3-culturedIL7RWT cells or IL-7-culturedIL7Rmutant Ba/F3 cells treated with SKi or DMSO for 72 h.gViability of leukemia cells from three independent mice, as compared to healthy B cell precursor controls in the presence of IL-7, cultured with increasing concentrations of SKi for 12 h. Viability index is normalized to the control condition (DMSO). Average ± s.e.m. is shown for each concentration.hViability (Annexin V/7AAD expression) of representative leukemia cells incubated with SK2 inhibitor Compound 55 (20 µM) or DMSO for 12 h.iDose-dependent effect of Compound 55 on leukemia cell viability (n= 4; 2 PAX5 P80R and 2 Ph-like).jCompound 55 in vivo administration scheme. Leukemic cells (2 × 105) were transferred into Rag−/−γc−/− hosts.kKaplan–Meier survival curves and respective log-rankpvalue of animals treated with vehicle (n= 7) or Compound 55 (n= 6; 5 mg/kg).l–nViability of mutantIL7Rhuman PAX5 P80R primary B-ALL cells cultured with increasing concentrations of (l) Dactolisib, (m) Compound 49, or (n) Compound 55 for 48 h. Viability index is normalized to the control condition (DMSO). Lines represent average of the duplicates, which are shown, for each patient sample. Source data are provided as a Source Data file. Enrichment plots were generated automatically by the GSEA software, while custom plots were generated using the ggplot2 R package. Immunoblotting Cell lysates were resolved by 12% SDS-PAGE and equal amounts of protein were transferred onto nitrocellulose membranes, and immunoblotted with antibodies against: p-STAT5 (Y694), p-S6(S235/236), p-Akt (S473), STAT5, S6 and Akt (Cell Signaling Technology), and β-actin (Santa Cruz Biotechnologies), as indicated in Supplementary Data 16 . Immunodetection was performed by incubation with horseradish peroxidase-conjugated secondary antibodies (Promega Corporation) and developed by chemiluminescence (Thermo Scientific; GE HealthCare). In vitro drug testing Leukemia cells were thawed and live cells magnetically sorted, according to the manufacturers’ instructions and specific alterations: we used an APC-conjugated Annexin V (invitrogen) to mark early/late apoptotic cells followed by secondary marking with anti-APC magnetic beads (Miltenyi Biotec), using Annexin V Binding Buffer (PromoKine). Cells were then cultured in duplicates as 10 6 cells/mL in IMDM GlutaMAX™ medium (supplemented with 10% FBS, 1% Pen/Strep, 1% MEM, 1% sodium pyruvate, 0.1% gentamicin, 0.1% β-mercaptoethanol) for the indicated time points in the presence or absence of the indicated concentrations of the Jak1/2 inhibitor INCB018424 (Selleckchem), the PI3K inhibitor LY294002 (Merck-Calbiochem), or the STAT5 small-molecule inhibitor Nʹ-((4-Oxo-4H-chromen-3-yl)methylene)nicotinohydrazide (Merck-Calbiochem). These inhibitors were added right after plating and dispensed in eight dilution steps using the D300(e) Digital Dispenser (Tecan). DMSO concentration was normalized to 0.4% in each well. Dilutions were done following a logarithmic distribution (INCB018424 and LY294002) or linear distribution (STAT5 Inhibitor). Cell viability was assessed at the indicated time points by flow cytometry analysis of forward scatter (FSC) versus side scatter (SSC) discrimination. The pharmacological inhibitors Sphingosine Kinase inhibitor (SKi) (Calbiochem), and compounds 49 and 55 (kindly synthesized by David R. Adams), the PI3K/mTOR inhibitor Dactolisib (BEZ235, NVP-BEZ235; Selleckchem), and the BET bromodomain inhibitor JQ-1 (Sigma Aldrich) were used to evaluate impact on cell viability. IL7R mut leukemia cells were thawed, and viable cells were either density-centrifuged using ficoll-paque or selected by Annexin V magnetic-activated cell sorting as described above. Cells were plated in a round-bottom 96-well plate as 10 6 cells/mL and incubated with increasing concentrations of sphingosine kinase pharmacological inhibitors or vehicle (DMSO). Human B-ALL diagnostic samples with IL7R type 1a mutations were previously collected from adult patients, at Saint-Louis Hospital, Paris, after informed consent. Patients were enrolled in GRAALL-2014 clinical trial (NCT02617004), approved by the French Comité de protection des personnes (CPP) and the Agence nationale de sécurité du médicament et des produits de santé (ANSM). BM mononuclear cells were isolated by Ficoll-paque gradient centrifugation and cryopreserved in liquid nitrogen. Thawed cells were treated as described above for mouse leukemia cells. For IL7R wild-type cells, control mice were sacrificed, and BM cells magnetically sorted for CD19 with anti-APC magnetic beads (Miltenyi Biotec) according to the manufacturer’s instructions. Cells were plated in a round-bottom 96-well plate as 10 6 cells/mL and incubated with increasing concentrations of SKi or vehicle (DMSO) and with IL-7 (1.25 ng/mL; Peprotech). Cell viability was measured using Annexin V/7AAD staining. Chemical screening We screened Ba/F3 cells stably transduced with human IL7R mutant for effects on viability (measured by Alamar Blue) using the 80 compounds included in the InhibitorSelect™ 96-Well Protein Kinase Inhibitor Library II (Calbiochem). Analysis of the screening results was performed with cellHTS2 R package [83] , where each replicate compound measurement was normalized using the negative controls (DMSO-control) and converted to a Z -score. Mutagenesis of murine Il7r gene The vector pUC19 harboring the wild-type murine Il7r cDNA (pUC19/Il7r WT) was used as template for mutagenesis, performed using the QuikChange II XL Site-Directed Mutagenesis Kit (Agilent Technologies) according to the manufacturer’s protocol. PCR amplifications were performed to introduce the p.S244_Val245insCPT using the mutagenic primer pair mIL7R-CPT-FWD and mIL7R_CPT_REV (Supplementary Data 17 ). The specific PCR conditions were the following: [denaturing phase 50 s at 95 °C; annealing phase 50 s at 60 °C; extension phase 5 min at 68 °C] × 18 cycles, thus generating the pUC19/ Il7r CPT. Mutagenesis was confirmed by Sanger sequencing. Ba/F3 cell culture Growth factor-dependent parental Ba/F3 cells or IL-7R-transduced Ba/F3 cells were maintained in culture medium (RPMI-1640 supplemented with 10% FBS, 2 mM l -glutamine, and penicillin/streptomycin). Parental Ba/F3 and Il7r WT transduced Ba/F3 cultures were supplemented with 2% (v/v) WEHI-3B-conditioned medium as source of murine IL-3 or 100 ng/mL of rhIL7 (Peprotech), respectively. Ba/F3 cells stably expressing wild type or mutant Il7r were deprived of IL-7 for 24 h prior the beginning of the experiments. Cells were then cultured in medium alone or supplemented with IL-7 (100 ng/mL) for the indicated time. Cell cycle analysis Cells (1–2 × 10 6 ) were resuspended in PBS, fixed and permeabilized with an equal volume of ice-cold 80% ethanol. Ribonuclease A (Sigma) was added at 50 mg/mL, and samples were incubated for 30 min at 37 °C. Propidium iodide (Sigma) was added at a final concentration of 2.5 mg/mL, and samples were analyzed by flow cytometry. Cell cycle distribution was determined using ModFit LT software (Verity). BrdU incorporation in vivo Mice were intraperitonially injected with 10 mg/mL BrdU (BD Pharmingen) and after 12 h BM was collected and cells stained with fluorochrome-conjugated anti-CD45, IgM, CD19, IgD, and B220 antibodies. Then, cells were stained with APC-conjugated anti-BrdU antibody and the DNA and 7AAD, using the BrdU Flow Kit (BD Pharmingen), according to the manufacturer’s protocol. MTS assay Cells were plated in a flat-bottom 96-well plate as 10 6 cells/mL for the indicated time points. MTS (3-(4,5-dimethylthiazol-2-yl)-5-(3-carboxymethoxyphenyl)-2-(4-sulfophenyl)-2H-tetrazolium; Promega) was then added to each well (20 µL/well), and cells were kept at 37 °C for 4 h. Absorbance was measured at 490 nm using the Infinite M200 microplate reader (Tecan). Construction of mutant Kras expression vectors The coding sequence of mutant murine Kras (Q61H) was PCR amplified from cDNA of spleen cells from an experimental mouse (from the model described above) harboring the Kras Q61H mutation using the forward and reverse primers described in Supplementary Data 17 . The PCR product was subsequently digested with Hpa I and Xho I (New England Biolabs) and cloned into the Hpa I and Xho I sited of pMIG (Addgene 9044). The clones were verified by Sanger sequencing. Retroviral production Retroviruses were produced using the pCLeco packaging vector and the pMig vector, either harboring the Q61H Kras mutation or mock, by co-transfection into HEK-293T cells, previously plated in a poly- d -lysine coating (Merck Life Sciences), using Lipofectamine 2000 (Life technologies) according to the manufacturer’s instructions. Subsequently, the viruses were concentrated using Amicon Ultra-15 Centrifugal Filter Unit with Ultracel-10 membrane from Merck Millipore and kept at −80 °C until usage. Retroviral transduction and transplantation of hematopoietic stem and progenitor cells IL7R mut and/or control mice were injected intraperitoneally with 300 μL of 5-fluorouracil (5-FU; 10 mg/mL), BM was collected 5 days after injection, and cells subjected to depletion of CD19 and CD3 with anti-APC magnetic beads (Miltenyi Biotec). Subsequently, cells were spin infected for 2 h at 1120 g at room temperature with 1 mL of viruses from either the pMig Kras Q61H or the pMig Empty vectors with 10 ng/mL of Polybrene (Merck Millipore). Rag2 −/− γ c −/− recipient mice were lethally irradiated (850 rad—two sub lethal irradiations) and reconstituted with 1.45 × 10 5 transduced cells and 2 × 10 5 stromal cells from Rag −/− γ c −/− mice. BM of recipient mice was analyzed 5 weeks after injection. Statistical analysis GraphPad Prism version 6-8.05 (GraphPad Software) was used to perform statistical analysis. Differences between groups were calculated using unpaired two-tailed t -tests. When appropriate, paired two-tailed t -tests and one-way ANOVA were used. Welsh’s correction was used in t -tests when variances were found different. Differences in the survival curves were calculated using log-rank Mantel–Cox test. P values lower than 0.05 were considered statistically significant. Tests used are indicated in figure legends. Reporting summary Further information on experimental design is available in the Nature Research Reporting Summary linked to this paper.